Mid-Pliocene warm-period deposits in the High Arctic yield insight into camel evolution The mid-Pliocene was a global warm period, preceding the onset of Quaternary glaciations. Here we use cosmogenic nuclide dating to show that a fossiliferous terrestrial deposit that includes subfossil trees and the northern-most evidence of Pliocene ice wedge casts in Canada’s High Arctic (Ellesmere Island, Nunavut) was deposited during the mid-Pliocene warm period. The age estimates correspond to a general maximum in high latitude mean winter season insolation, consistent with the presence of a rich, boreal-type forest. Moreover, we report that these deposits have yielded the first evidence of a High Arctic camel, identified using collagen fingerprinting of a fragmentary fossil limb bone. Camels originated in North America and dispersed to Eurasia via the Bering Isthmus, an ephemeral land bridge linking Alaska and Russia. The results suggest that the evolutionary history of modern camels can be traced back to a lineage of giant camels that was well established in a forested Arctic. Today, camels ( Camelus , Camelini) are known from arid regions that extend from northern Africa to the Asian interior. Their nearest living relatives are llamas, alpacas, vicuñas and guanacos (Lamini) of South America. The family Camelidae originated in North America during the Eocene period (~45 Ma) and diversified in the early Miocene, giving rise to at least 20 genera [1] . The modern tribes Lamini and Camelini, diverged from one another by about 17 Ma in the Early Miocene [1] . Subsequently, Camelini had reached Eurasia by the Late Miocene, whereas Lamini dispersed to South America about 3 Ma. Paracamelus, the likely ancestor of Camelus, is known from the fossil records of Asia, Europe and Africa, the oldest known members being from Spain (Vento del Moro; ca 7.5–6.5 Ma) [2] and China [3] . The North American lineage most closely related to the Paracamelus + Camelus clade is debated, with possible candidates including Megacamelus, Procamelus , and Megatylopus [1] , [2] , taxa all only known from localities south of 45°N. In the Yukon, rare fossil remains of a giant camel, collected from Plio-Pleistocene deposits of the Old Crow Basin at ~67°N, are considered cf. Paracamelus N [4] . The first giant Yukon fossil camel specimen, a proximal phalanx, was discovered in 1913 (ref. 5 ). Since then isolated bones, including ankle elements, partial long bones and teeth, have been collected. Most of these bones are from the famous ‘supermarket’ for bones at Old Crow Locality 11A. That locality, a gravelly point bar, produced hundreds of fossils extending at least from Early Pleistocene to Holocene age. One bone (astragalus) was excavated from the basal clay unit at Old Crow Locality 44 [6] (ref. 6 ). The stratum bearing the camel bone is clearly older than last interglacial age, perhaps Early to Middle Pleistocene. Before the discovery of the High Arctic fossil material reported here, the Yukon giant camel was the most northerly recorded cameline, and showed that populations of the Paracamelus lineage had extended at least as far North and East as Beringia. The discovery of camel remains from Ellesmere Island, identified with the help of collagen fingerprinting, provides surprising new insight into the evolutionary history of camels. The Ellesmere camel is the most northerly evidence of camels and it inhabited the High Arctic during the mid-Pliocene warm period when the area was forested and the broad channels of the western Canadian Arctic Archipelago (CAA) were filled with sediment. Terrestrial cosmogenic nuclide burial dating indicates the camel existed >3.4 Ma ago. The findings provide evidence for understanding the evolutionary history of a lineage that also gave rise to modern camels. Geological context Unconsolidated late tertiary stream deposits are found throughout the CAA. These deposits comprise bedded sands and pebble gravels, interbeds of organic detritus and subfossil wood, and centimeter-to-metre-thick peat beds. The deposits are thickest in the western CAA, where the Pliocene Beaufort Formation unconformably overlies the Miocene Ballast Brook Formation [7] , [8] . Where preserved, the upper surfaces of the stream deposits are typically parallel to the uppermost bedding, and generally dip gently westward towards the Beaufort Sea and Canada Basin. The deposits have been interpreted as a once continuous and extensive wedge of clastic sediments that extended offshore, but which are now abandoned, incised and isolated by large channels that separate the islands of the CAA. In the High Arctic, particularly Ellesmere Island, high terrace fluvial gravels and sands with interbedded peat deposits are regarded as having been formed in a contemporaneous but more continental depositional environment than the Beaufort Formation coastal plain [7] . Until now there was no chrono-stratigraphic means of linking the Beaufort Formation and the Ellesmere high terrace deposits. We focus on two high terrace gravel sections—the Beaver Pond (BP) site and the nearby Fyles Leaf Beds (FLB) site that were previously discovered and studied by others [9] , [10] , [11] , [12] . Exposed on a cliff section at the BP site is a >20 m succession of fine to coarse cross-bedded fluvial sands conformably overlain by cobble gravels interpreted to be glacial outwash and capped by 2 m of till ( Fig. 1 ). The section rests on the northeastern edge of an interfluvial plateau south of Strathcona Fiord. The till and proximity of the site to nearby extant ice caps implies that during multiple glaciations glacier ice covered this part of the terrace and likely eroded from the top of the section an unknown thickness of deposit (but <30 m based on topographic projection over the entire 20 km terrace surface). A peat deposit, up to 2.4 m thick, situated within the fluvial sand unit, is characterized by exceptionally well-preserved plant, invertebrate and vertebrate remains [13] . The plants are subfossil in preservation, and bear evidence of a boreal-type forest and wetland [13] . The BP site has also yielded a rich Pliocene vertebrate fauna, including the remains of various carnivores as well as beaver, horse, rabbit and deerlet [10] , [13] . Palaeotemperature estimates for the FLB and BP sites, using multiple proxies, suggest a mean annual temperature for the area of −1.4±4.0 °C, 18.3±4.1 °C warmer than present, with a significantly warmer winter [12] , [14] . A large boulder on the till surface has a minimum. 10 Be exposure age of 78.9±7.0 ka (1σ), and the moderate soil development in the till is consistent with a late Pleistocene age. 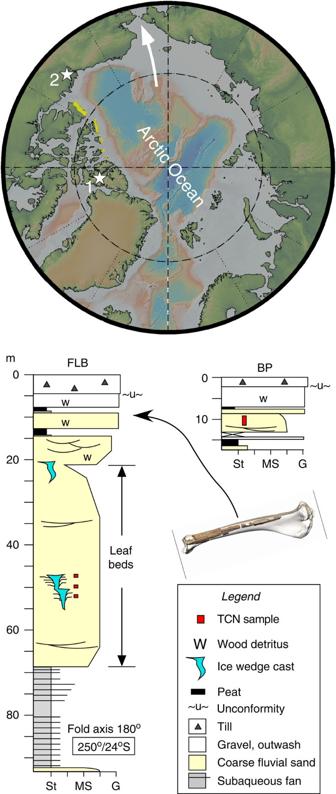Figure 1: Arctic circle and fossil sites. Locations (white stars) of fossil areas yielding the remains of Arctic giant camels are shown. Location 1.Fyles Leaf Bed (FLB) and Beaver Pond (BP) sites, Strathcona Fiord, Ellesmere Island, Nunavut;Location 2.Old Crow Basin, Yukon Territory. Grey shaded bathymetry indicates <100 m water depth. Yellow shading is current distribution of Beaufort Formation19. Schematic stratigraphic columns for the FLB and BP sections showing TCN sample depths and location of the source of the Camelini fossil fragments. St, silt; MS, medium sand; G, gravel. Figure 1: Arctic circle and fossil sites. Locations (white stars) of fossil areas yielding the remains of Arctic giant camels are shown . Location 1. Fyles Leaf Bed (FLB) and Beaver Pond (BP) sites, Strathcona Fiord, Ellesmere Island, Nunavut; Location 2. Old Crow Basin, Yukon Territory. Grey shaded bathymetry indicates <100 m water depth. Yellow shading is current distribution of Beaufort Formation [19] . Schematic stratigraphic columns for the FLB and BP sections showing TCN sample depths and location of the source of the Camelini fossil fragments. St, silt; MS, medium sand; G, gravel. Full size image The FLB site refers to a ~1-km long natural exposure of >90 m of Beaufort Formation-equivalent high-terrace deposits, located 10 km south of BP ( Fig. 1 ). The base of the section exposes steeply-dipping finely-laminated silt and fine sand that were deposited in a shallow nearshore lake or marine deltaic environment. These sediments coarsen up into a 55 m thick succession that comprises more than one thousand, fining upward layers of ripple cross-laminated sand. The layers are ~3 cm thick, can be traced laterally for >100 m, and most terminate with a compressed layer of well-preserved sub-fossil moss and leaves. The succession may represent a fluvial braided system with an annual breakup flood deposit covered with reworked fallen leaves, and hence, represents only a millennium or two in its entirety. Syn-depositional fossil thermal contraction features (‘ice wedge casts’ observed at 25 and 50 m depth, Fig. 1 ) within this unit indicate that conditions were colder than those represented at the BP site peat layer [15] , and probably reflect the temporal variability in palaeoclimate recorded at these neighbouring sites. Overlying a sharp conformable contact is a sequence of trough-cross bedded coarse sandy gravel beds that contain interbeds of woody detritus and mossy autochthonous peats. The sequence is capped by dissected glacial outwash and till. The peat deposits near the top of the FLB exposure appears similar in elevation to those of the BP fossil site (~400 m). The camel fossil material, representing the first vertebrate fossil from the FLB site, was recovered over three field seasons (2006, 2008, 2010) from a steeply-sloping (>30°) colluvial surface. The fossil-bearing colluvium extended over 12 m vertically, from a point source located at or just above a mossy peat layer, in the upper levels of the section ( Fig. 1 ). Roughly, 30 fragments were recovered, varying in size from 1.4 to 7 cm, along the longest axis. Age estimates for the high terrace gravel We used the terrestrial in situ cosmogenic nuclide (TCN) burial dating method [16] to provide the first direct age estimates for both the FLB and BP fossil sites ( Fig. 2a ). Cosmogenic 26 Al and 10 Be are produced in quartz exposed to secondary cosmic rays within a few tens of metres below the Earth’s surface. Once buried and shielded, the ratio of the nuclides changes due to differences in their decay rate. A series of four 2 kg quartz-rich samples were collected from coarse sand at BP a few metres above the main peat layer. Because there is no evidence of a soil or unconformity between the two sites, the difference between the age of the peat and adjacent TCN samples is well within the ~10% 1 σ error of the TCN method. At the FLB site, a sample was dated within the rhythmically bedded sandy leaf beds, ca 40 m below correlative peat beds and the camel fossil ( Fig. 1 ). The time represented by the sand layers separating the peats from the samples is negligible compared with the uncertainty of burial dating. We assume the quartz sand acquired a 26 Al/ 10 Be that reflected a simple shallow exposure history before deposition. A simple history is justified on the grounds of isotope chemistry and topography ( Supplementary Methods Geochronology ). Although we are unable to correct for the potential effect of post-burial TCN production by muons, because the burial depth has most certainly varied and therefore the burial ages are minima, the isotope results indicate that post-muonic production may also be negligible ( Supplementary Fig. S1 ). 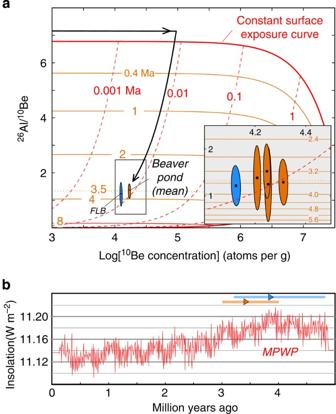Figure 2: Geochronology of Ellesmere camel. (a)26Al/10Be versus log10Be plot for the five samples collected for burial dating. Black arrow illustrates a simple exposure history (minimum exposure duration indicated by dashed red lines) followed by instantaneous burial (minimum burial durations indicated by solid brown lines). Blue: Beaver Pond Site and Orange: Fyles Leaf Beds Site. The weighted mean age for all four samples of the Beaver Pond Site (shown in inset) is provided in the main graph. This graph assumes no muonic production, as discussed in text (cf.Supplementary Fig. S2). (b) Mean insolation at 78.55 N latitude for winter season (270–0 degrees from vernal) symmetrically smoothed (25 pts) with simple moving window averaging using FFT43,44. The maximum-limiting and minimum-limiting ages with 1 σ total error bars are shown above. MPWP, Mid-Pliocene Warm Period; FFT, Fast Fourier Transform. Figure 2: Geochronology of Ellesmere camel. ( a ) 26 Al/ 10 Be versus log 10 Be plot for the five samples collected for burial dating. Black arrow illustrates a simple exposure history (minimum exposure duration indicated by dashed red lines) followed by instantaneous burial (minimum burial durations indicated by solid brown lines). Blue: Beaver Pond Site and Orange: Fyles Leaf Beds Site. The weighted mean age for all four samples of the Beaver Pond Site (shown in inset) is provided in the main graph. This graph assumes no muonic production, as discussed in text (cf. Supplementary Fig. S2 ). ( b ) Mean insolation at 78.55 N latitude for winter season (270–0 degrees from vernal) symmetrically smoothed (25 pts) with simple moving window averaging using FFT [43] , [44] . The maximum-limiting and minimum-limiting ages with 1 σ total error bars are shown above. MPWP, Mid-Pliocene Warm Period; FFT, Fast Fourier Transform. Full size image The four BP samples yield a weighted mean date of > Ma (1 σ total error, the small but unknown muonic contribution means that this is a minimum age), which provides a minimum limiting age for the associated fossil-bearing peat ( Supplementary Tables S3 and S4 , Supplementary Methods Geochronology ). The single sample at the FLB site provides a minimum age for the overlying peat and camel-bearing layer of Ma. These ages fall within the mid-Pliocene warm period ( Fig. 2b ). In particular, the ages correspond to the general maximum in mean winter season insolation delivered at the latitude of the camel site throughout the Neogene, consistent with the palaeotemperature data and apparent presence of only discontinuous permafrost. The TCN age at FLB is from sediment adjacent to ice wedge casts ( Fig. 1 ), which provides the northern-most dated evidence of Pliocene thermal contraction cracking. These high terrace ages also validate previous fossil mammal [13] and floral biostratigraphic correlation with the Beaufort Formation, numerically and palaeomagnetically dated on Meighen Island with amino-acid racemisation and Sr-isotopes in mollusks to ~3 Ma [18] . We suggest that the high terrace gravel generally grades westward to the Beaufort Formation palaeo-landscape surface, connecting to the broad clastic wedge that covered the western edge of the CAA and the currently submerged Iperk Formation [18] , [19] . The camel remains were found in sands from just above the dated sands at the FLB site ( Fig. 1 ), suggesting that when the camel lived, Ellesmere Island and the rest of the CAA region was a largely continuous land mass. In addition, the ages for the top of the high terrace gravel provide a constraint on the cessation of Beaufort Formation deposition, and the timing of its widespread incision. This is consistent with the general timing of the initiation of glaciation in North America at the Plio-Pleistocene boundary [20] , and the consequent drop in sea level, which led to stream incision. Ellesmere Island fossil The Ellesmere Island fossil camel specimen NUFV (Nunavut Fossil Vertebrate) 210 is housed at the Canadian Museum of Nature. The specimen forms part of the lateral surface of a large tibia. The fragments making up the tibia were scanned using an Arius three-dimensional surface scanner and assembled digitally ( Fig. 3a ). The specimen preserves two distinguishing characters. The first is a large nutrient foramen, characteristic of mammal tibiae. The second is the proximal rim of the fibular notch, which implies the presence of a malleolar bone (fibula remnant), characterizing ruminant artiodactyls, such as deer, cows and camelids [21] . Due to the fragmentary preservation, no standard morphometric measurements could be acquired. The morphology alone is not sufficient to confidently identify the artiodactyl as a cameline; however, the large size is highly suggestive. In the late Neogene of North America, the largest artiodactyls by far are the camelines [22] , suggesting that the Ellesmere artiodactyl specimen most likely represents a member of Camelini. Camelini includes the living camels ( Camelus ), their probable ancestor the Eurasian Paracamelus , multiple North American fossil forms, Procamelus , Titanotylopus, Megatylopus , Megacamelus and Gigantocamelus [1] , as well as the Yukon giant camel (cf. Paracamelus ) [4] . 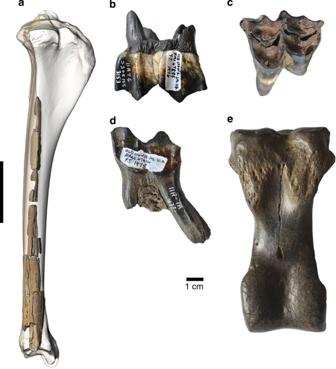Figure 3: Fossil remains of Arctic giant camelines. (a)Lateral view of right tibia specimen (NUFV 210), from FLB site, Strathcona Fiord (Ellesmere Island), shown within the tibia of an extant camel (Camelus dromedaries,ROM MAM 94191). The modernCamelustibia has been scaled up 30% to match the size of the fossil tibia. Scale bar, 10 cm. (b,c) Lateral and occlusal view of upper left second molar of Yukon camel (CMN 47895). (d) Medial view of lower right second (?) molar of Yukon giant camel (CMN 47914). (e) Posterior view of first proximal phalanx of Yukon giant camel (CMN 48074). Figure 3: Fossil remains of Arctic giant camelines. (a) Lateral view of right tibia specimen (NUFV 210), from FLB site, Strathcona Fiord (Ellesmere Island), shown within the tibia of an extant camel ( Camelus dromedaries, ROM MAM 94191). The modern Camelus tibia has been scaled up 30% to match the size of the fossil tibia. Scale bar, 10 cm. ( b , c ) Lateral and occlusal view of upper left second molar of Yukon camel (CMN 47895). ( d ) Medial view of lower right second (?) molar of Yukon giant camel (CMN 47914). ( e ) Posterior view of first proximal phalanx of Yukon giant camel (CMN 48074). Full size image In order to estimate the relative size of the fossil specimen, it was compared with modern dromedary ( Camelus dromedarius ) and Bactrian camel ( Camelus bactrianus ) tibiae. The modern specimens were also visualized using computed tomography (CT) to allow for cortical thickness comparisons. Informed by the cortical thickness and surficial dimensions the Ellesmere tibia is estimated to have been approximately 575 mm in length, 29% larger than that of modern camels ( Fig. 3 , Supplementary Fig. S2 , Supplementary Table S1 ). From the size of the tibia, the Ellesmere camel was comparable in body size to other giant camels within Camelini, such as the Asian Paracamelus gigas and the Yukon giant camel (see Fig. 3b–e and Supplementary Table S2 ). Collagen fingerprinting and bone preservation Although the fossil bone (NUFV 210) recovered from the FLB site was highly fragmentary and incomplete, we were able to use the surviving collagen to help confirm its taxonomic identity. Type I collagen, the dominant protein in bone which is shown to survive longer than other genetically informative biomolecules [23] , is sufficiently variable between mammal genera to be useful taxonomically [24] . We analysed bone fragments from each of the three collection years using methods modified from Buckley et al . [24] (see Methods). The results were compared with a database of genus-specific collagen peptide markers from 37 terrestrial mammal species ( Supplementary Methods ) and most closely matched the camel, C. dromedarius . For further comparison, additional camelids were also analysed, including samples of modern C. bactrianus , alpaca ( Lama pacos) , llama ( Lama glama ) and fossil camelids, including three Late Neogene specimens from the North American midwest ( Titanotylopus nebraskensis, Megatylopus gigas, Gigantocamelus), two from the Yukon (cf. Paracamelus ) and one Pliocene Paracamelus specimen from Mongolia. Of the additional fossils, only the Yukon specimens yielded collagen. Peptide markers for the llama and alpaca matched those already described for the vicuña elsewhere [24] making it possible to identify markers for the Lamini sub-family ( Supplementary Information ). In the three known Camelini specimens (Yukon camel, Bactrian and dromedary camel), markers for the Camelini sub-family [24] were present ( Fig. 4β ). Although a number of potentially diagnostic peaks were present, only one of these ( Fig. 4α ) could be confidently shown to represent homologous collagen peptides useful for distinguishing between the two extant species ( Fig. 4 ); the homologous Yukon giant camel peptide matched that of the dromedary camel. The analysis of the Ellesmere camel fossil, carried out as the first collagen analyses in a new laboratory to avoid any possibility of contamination, was found it to be nearly identical to the dromedary and Yukon camel. The observed relative amount of collagen peptide-bound glutamic acid (Q) deamidation in this peptide ( Fig. 4 , inset), a particularly slow-rate reaction, is in agreement with its antiquity. The survival of >3.4 Ma collagen is exceptional, but consistent with the cold thermal history of the site, conducive to biomolecular preservation [25] . These sub-zero temperatures not only slow reaction rates, but also likely lock reactant fluids up as ice, temporarily dehydrating the specimens and further reducing diagenetic rates of reaction. 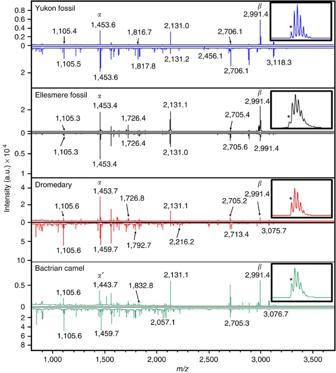Figure 4: Collagen spectra of modern and fossil Camelini. Ellesmere fossil camel (NUFV 210), Yukon fossil camel (CMN 48096),Camelus bactrianus,Camelus dromedarius. ‘α’ denotes homologous peptides (Supplementary Fig. S4), modified in the Bactrian camel (α′); ‘β’ denotes one of the most intense species markers, shared by all camelines analysed here, observed atm/z2,992 representing the peptide sequence GPSGEAGTAGPOGTOGPQGLLGAOGFLGLOGSR, where O=Hyp and the Q is deamidated (Supplementary Fig. S5). Insets show the isotopic envelopes for peptide ‘β’ (with the monoisotopic peak marked with an asterisk), within which the effect of increased Q deamidation in the ancient peptides can be observed. Figure 4: Collagen spectra of modern and fossil Camelini. Ellesmere fossil camel (NUFV 210), Yukon fossil camel (CMN 48096), Camelus bactrianus , Camelus dromedarius . ‘ α ’ denotes homologous peptides ( Supplementary Fig. S4 ), modified in the Bactrian camel ( α ′); ‘ β ’ denotes one of the most intense species markers, shared by all camelines analysed here, observed at m / z 2,992 representing the peptide sequence GPSGEAGTAGPOGTOGPQGLLGAOGFLGLOGSR, where O=Hyp and the Q is deamidated ( Supplementary Fig. S5 ). Insets show the isotopic envelopes for peptide ‘ β ’ (with the monoisotopic peak marked with an asterisk), within which the effect of increased Q deamidation in the ancient peptides can be observed. Full size image Fragments of NUFV 210 were also analysed by Field Emission Gun-Environmental Scanning Electron Microscope (FEG-ESEM) to provide geochemical details of preservation. 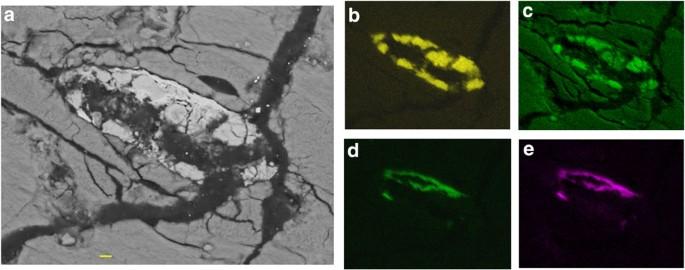Figure 5: FEG-ESEM maps of a cross-section of Ellesmere fossil camel bone. Maps showing a Haversian canal infilled with mineral precipitates. (a) Back-scattered electron image. X-ray maps are also shown: (b) Fe, (c) O, (d) Ba, (e) S, lighter colours indicate higher concentrations of the element. (Scale bar, 2 μm. Width of all images approximately 50 μm.) Elemental distributions within the canal are consistent with iron oxyhydroxide and barium sulphate precipitation. Figure 5 shows that at least two mineral phases have precipitated from aqueous fluids both infilling and coating the bone (hydroxyapatite) surfaces. Iron and oxygen maps indicate iron oxyhydroxides, whereas barium and sulphur show the presence of barytes (BaSO 4 ). These secondary precipitates are both indicative of relatively oxidizing conditions. ESEM images of an unprepared bone surface also show an extensive coating of micro-crystalline mineral precipitates including barytes, iron oxyhydroxides and rare-earth element enriched apatite. Phyllosilicate grains derived from the embedding sediments are also present. Staining appears continuous on the bone surface, lacking obvious evidence of long-distance fluvial transportation, and thus supporting in situ oxidation at the FLB site. Figure 5: FEG-ESEM maps of a cross-section of Ellesmere fossil camel bone. Maps showing a Haversian canal infilled with mineral precipitates. ( a ) Back-scattered electron image. X-ray maps are also shown: ( b ) Fe, ( c ) O, ( d ) Ba, ( e ) S, lighter colours indicate higher concentrations of the element. (Scale bar, 2 μm. Width of all images approximately 50 μm.) Elemental distributions within the canal are consistent with iron oxyhydroxide and barium sulphate precipitation. Full size image The fine-grained coating of precipitates has decreased the porosity and permeability of the bone and could have acted to seal pockets of organic matter from aerobic degradation, thus enhancing preservation [26] . ESEM analysis also resolves extremely carbon-rich areas, which likely represent organic matter, probably including the retrievable collagen. The unique combination of relatively low temperatures (compared with other mid-latitude specimens that failed collagen analysis in this study) and secondary precipitation acted in concert to allow biomolecular longevity in the Ellesmere Island burial environment. Evolutionary inferences Given that the collagen fingerprinting, in combination with evidence for large body size, suggests that the Ellesmere camel and the giant Yukon camel are near relatives, we can benefit from the Yukon camel record, which includes dental and postcranial evidence, typically regarded as important for inferring evolutionary relationships. The Yukon camel shows morphological similarities with some North American giant camels and also the Eurasian Paracamelus . In particular, the upper molars of the Yukon camel have well-developed styles and ribs ( Fig. 3b–d ), a characteristic shared with Paracamelus [2] , Megacamelus+Gigantocamelus [1] , [27] , and at least some Megatylopus species. All of the North American taxa ( Titanotylopus, Megatylopus , Megacamelus and Gigantocamelus) have high-crowned molar (hypsodont) teeth, with Megatylopus being the least hypsodont [27] . In modern camels, the teeth are even less hypsodont than in Megatylopus [28] . Hypsodonty in mammals is a specialized condition, and once acquired within a lineage it is usually, if not always, retained [29] . So the appearance of relatively lower crowned teeth within Camelus suggests that its ancestor had low-crowned teeth, implying that the North-American mid-latitude camels ( Procamelus , Megacamelus , Gigantocamelus and Megatylopus) are too dentally specialized (too hypsodont) to be ancestral to the lineage that gave rise to Camelus . Molar hypsodonty measurements require unworn, or little worn molars, usually of the lower third [30] or the upper and lower second molars [31] . Hypsodonty estimates are currently unavailable for the Yukon camel and Paracamelus . However, it is notable that in the Eurasian Paracamelus [2] and the Yukon camel ( Fig. 3 ), the molar roots are extremely well developed, emerging from a thick dentine base, which forms a dentine surface around the tooth. In more hypsodont camels (e.g., Procamelus , Megacamelus ), the root area is relatively less well developed. Teeth develop from apex to root, and comparative evidence suggests that increased crown height occurs at the expense of the root area, resulting in smaller roots [32] . The extremely well-developed roots of the Yukon camel and the Eurasian Paracamelus , suggests that these forms were relatively low-crowned, as would be expected of Camelus near-relatives. The size and morphology of the first phalanx also suggests close affinities between the Yukon camel and Paracamelus . In camels, the morphology of the proximal region of the plantar surface is recognized as phylogenetically informative [27] , [33] . Rugosities in this area provide attachment for the ligaments of the proximal sesamoids. In turn, the sesamoids serve as the main attachment area for the interosseous musculature. Although, the basic proportions of the Yukon camel first phalanx are similar to those of Gigantocamelus spatulus (following the taxonomy of Honey et al . [1] ), in Paracamelus [2] and the Yukon camel the ligament scar is more pronounced and the centre of the ligament scar forms a deeply entrenched V-shaped notch that opens distally ( Fig. 3e ). In Gigantocamelus spatulatus [33] and Megacamelus merriami [27] , the scar forms two triangular patches on either side of a slightly recessed region. At least one individual of Megatylopus gigas also shows a deeply entrenched V-shaped notch, however, the overall proportions of the phalanx are much more gracile in Megatylopus than in Paracamelus or the Yukon camel. In modern Camelus, the morphology differs: the centre of the ligament scar is raised. Overall, the phalangeal morphology is most similar between the Eurasian Paracamelus and the Yukon camel, supporting phylogenetic affinities. The discovery of giant camel remains on Ellesmere Island extends the range of North-American camels northward by ~1,200 km. The Ellesmere camel is the first evidence that camels inhabited the High Arctic at a time when global temperatures were ~2 to 3 °C greater than modern. Palaeoenvironmental reconstruction of the upper portions of the FLB and BP fossil sites suggests that during relatively warmer times in the mid-Pliocene the Strathcona Fiord area of Ellesmere Island supported a larch dominated forest habitat, with a slightly below freezing mean annual temperature. Yet, cooler mid-Pliocene conditions allowed for thermal contraction cracking (ice wedges). Thus, it is likely that the Ellesmere camels survived winters with very low temperatures and ~6 months of 24-h darkness, perhaps inhabiting the forest-tundra ecotone. Although their localities are over 2,000 km apart, the Ellesmere Island and Yukon camels show nearly identical collagen fingerprints (shared also with the modern dromedary). The similarities are striking when compared with the differences observed between the two living camel species ( Fig. 4 ), and suggest that the Arctic fossils represent closely related populations, possibly the same species. The North-American Arctic cameline shows morphological affinities with Paracamelus , but lived long after the appearance of Paracamelus in the mid-latitudes of Eurasia, 6–7 Ma. It is likely that Arctic camels were originally part of a Miocene arctic biotic province that intermittently or continuously spanned the Bering Isthmus. In the late Miocene, Beringia probably supported a mixed coniferous boreal-type forest, perhaps bordered by steppes [34] , [35] . The concept of an Arctic biotic continuity is supported by the mammalian fossil record (largely south of 55°N), which records numerous Miocene ‘dispersal events’ between Eurasia and North America [35] , [36] . The terrestrial Arctic biotic continuity would have been broken ~5.5 Ma when tectonic rifting led to the opening of the Bering Strait [37] ( Fig. 1 ). Evidence of an oscillating or possibly continuously collapsed Pliocene West Antarctic ice sheet [38] and high Pliocene sea levels [39] , [40] suggest that from 5.5 to ~3.0 Ma the Beringian land mass was often, if not always, submerged, hindering intercontinental dispersal of terrestrial organisms. Populations may have dispersed across the Bering Strait in cold winters via Arctic sea ice. Year round dispersal could have ensued at times during the Pleistocene, when sea levels were significantly lowered periodically due to continental glaciation and the Bering Isthmus had re-emerged. The appearance of the Paracamelus lineage in the Yukon during the Pleistocene (2.6 – 0.01 Ma) and mid-Pliocene High Arctic (~3.5 Ma), suggests that populations of this lineage were living in the North-American Arctic for >7 Ma. It is likely that modern camels are derived from a lineage (that is, ‘ Paracamelus’ ) that was originally adapted to living in Late Neogene, northern forests, and some traits seen in modern camels may reflect this heritage. For example, modern camels are characterized by cheek teeth with relatively low crowns compared with North-American mid-latitude fossil camels [28] (see above). In ungulates today, lower crowned teeth characterize taxa that inhabit more closed, forested, habitats, whereas higher crowned teeth are associated with open habitats [29] . So the relatively low-crowned teeth seen in camels today may be the result of a forest-dwelling ancestor. Other specialized traits seen in modern camels may also have served well in an Arctic realm. For example their wide flat feet function well on soft substrates, such as sand or snow. Their iconic hump(s), containing fat, also may have been adaptive. As seen in high-latitude ungulates today [41] , fat deposits could have been critically important for allowing populations to survive and reproduce in harsh climates characterized by 6-month long, cold, winters. Geochronology TCN burial dating [16] with cosmogenic 10 Be and 26 Al was conducted at the Dalhousie Geochronology Centre on five samples of coarse sand from the two fossils sites. In 2008, four samples (SF-08-C-001 to SF-08-C-004) were collected in a vertical sequence in cross-bedded fluvial sand beds from 8.7–10.4 m below the uppermost surface of the till cover at the BP site, a few metres stratigraphically above the well-known and thickest BP peat layer. Also in 2008, three sand samples (SF-08-C-015 to SF-08-C-017) were collected from the 90 m FLB site section at 38 m depth below the till surface. (The 26 Al/ 27 Al of sample SF-08-C-016 was smaller than the blank and the Inductively Couple Plasma-Optical Emission Spectrometer (ICP-OES) measurement of Al in sample SF-08-C-017 failed an internal consistency check, so these samples are not included in the remaining discussion.). The sands were up to 75% quartz but also contained a significant fraction of garnet, so Franz magnetic separation was used to initially purify the samples. This was followed by rinsing, 2 h in boiling aqua regia in Teflon beakers and 15 min in 2:1 hydrofluoric acid (HF): 18 MΩ deionized water. We used the 250–355 μm fraction. After drying and weighing, the samples were subjected to an additional 2 days with four cycles of ultrasonification in dilute HF acid and rinsing in type 1 deionized water to ensure that more than 30% of the quartz had dissolved to remove meteoric 10 Be [42] . Quartz purity was verified by microscopy and with an Al test for the presence of feldspar (ensuring less than 100 p.p.m. Al in 1 g of sample, using Quant-EM Al strips). Very few inclusions were noted in the quartz. After drying and thermal equilibration, ~150 g of the pure quartz samples were weighed in 300 ml Teflon digestion vessel (sample SF-08-C-003 had only 120.7010, g). Approximately 0.20 g of 985±21 μg ml −1 Be carrier (Be-Carrier3-bottle2, density 1.013 g ml −1 , 1 σ uncertainty is based on more than one dozen ICP-OES and ICP-Mass Spectrometers at four institutions within 2 years of this experiment) was added to each sample. This carrier was prepared by J. Klein from a beryl recovered deep within the Homestake Goldmine in South Dakota, and has an average 10 Be/ 9 Be of 4 × 10 −15 as measured at U. Penn and LLNL Accelerator Mass Spectrometry (AMS) facilities. After initial dissolution in Trace Grade HF and in the presence of Trace Grade perchloric acid, the samples were converted to chlorides, brought to 100 ml in 2% hydrochloric and 10 ml aliquots were removed to measure the native Al abundance. Enough Al carrier (SPEX 1,000 μg ml −1 ICP-MS standard) was added, depending on the estimates of Al in the quartz from the Quant-EM strips, to optimize Al 2 O 3 targets for AMS (~4 mg of Al). The anion and cation column chemistry with 10 and 19 ml of Bio-Rad resins, respectively, in 50 ml glass columns with fritted discs were separated with controlled precipitations using high purity ammonium hydroxide, we precipitated the metal hydroxides with ultrapure (99.999%) ammonia gas. The hydroxides were ignited in quartz vials in a Bunsen flame for at least 1 min after turning white. The Be (and Al) oxides were mixed with equal amounts of niobium (and silver) by volume, and packed into stainless steel target holders from LLNL that were cleaned thoroughly with Citronex and Nitric Acid. Dating of the single granitic boulder (SF-08-C-014, maximum height=0.8 m) on till (sample thickness=3 cm from broad low-gradient peak) followed the same chemistry procedure, except only 25 g of pure quartz were used and 26 Al was not measured. The 10 Be blanks were elevated ( 10 Be/ 9 Be=1.29 × 10 −14 ) relative to the carrier, which we have observed from previous experiments that required high volumes of acids for dissolution of the large masses. The 10 Be currents (5–9 μamp) were less than the standard (07KNSTD3110, 20–22 μAmp). Boron isobaric corrections for the 10 Be/ 9 Be were ~1% for the BP samples but 3.2% for the FLB site sample (SF-08-C-016), suggesting that the latter may have experienced boron contamination just prior to loading. The 26 Al blanks were normal ( 26 Al/ 27 Al=2.37 × 10 −15 ) and currents on all samples were double (1.5 versus 0.8 μAmp) that of the standard (KNSTD10650). Because such a large sample mass was used, the blank corrections were less than a few percentage and did not contribute significant error. The AMS precisions on the quartz samples averaged 2.7% for 10 Be but 32% for 26 Al, owing to the extremely low abundance of 26 Al. The reduced data are provided in Supplementary Table S3 . One-sigma precision in the ICP-OES measurement of native Be and Al in solution by MAXXAM Analytics was reported to be approximately 5%, however, this may be an underestimate. The total 1 σ uncertainty in the measured 26 Al/ 10 Be was calculated by adding in quadrature the AMS precisions, ICP error and a 2% error in geochemistry mainly controlled by uncertainty in carrier concentrations. The burial ages for the samples are provided in Supplementary Table S4 . The calculated age of the sample at the FLB site is 3.7 +1.0/−0.7 Ma. Size estimation To estimate the relative size of NUFV 210 (a lateral margin of a right tibia), the distance between the top of the fibular notch and the nutrient foramen in the fossil was compared with that of C. bactrianus and C. dromedarius ( Supplementary Fig. S1 , Supplementary Table S1 ). The small gap seen in the assembled fossil ( Fig. 2 , Supplementary Fig. S1 ) is 6 mm, equivalent to the length of a sample that was removed in a preliminary phase of the study. However, it is possible that more bone is missing. Therefore, the size estimation, based on length, is regarded as a minimum estimate. Size was also estimated using the cortical thickness of NUFV 210 by comparing measurements of the fossil cortical thickness, with CT scans of the modern specimens of C. bactrianus and C. dromedarius ( Supplementary Fig. S1 , Supplementary Table S1 ). CT scanning as at the Montfort Hospital (Ottawa, Canada). Collagen analysis To extract collagen from the fossil specimens, the bone fragments were sampled using a fresh diamond-tipped dremel drill. Approximately 0.1–0.2 g of collected bone powder was then demineralized for 18 h using 0.6 M hydrochloric acid, leaving an acid-insoluble collagen pellet upon centrifugation at 13,000 g. This predominantly collagenous pellet was gelatinized at 70 °C for 4 h in 0.5 ml of 50 mM ammonium bicarbonate (pH 7.8), and the supernate concentrated (30 kDa molecular weight cut-off (MWCO); GE Healthcare) before tryptic digestion (2 μg; Promega) overnight at 37 °C. The samples were then acidified to 0.1% trifluoroacetic acid (TFA) and further concentrated using C18 ziptips (OMIX) into two fractions, 0–10% acetonitrile (ACN) in 0.1% TFA and 10–50% ACN in 0.1% TFA [24] . The samples were then evaporated and resuspended in 10 μl 0.1% TFA before matrix-assisted laser desorption/ionization (MALDI)-mass spectrometer (MS) analysis. One microlitre of each fraction was spotted onto a Bruker Ultraflex 386-well MALDI target plate (Bruker) and co-crystalized with 1 μl of α-cyano hydroxycinnamic acid (Fluka) solution (1% (wt/vol) in diluent=50% ACN, 50% H 2 O, 0.1% TFA), which was applied to the sample spot while still wet and allowed to air dry. The target plate was then loaded into a calibrated Bruker Ultraflex II MALDI–time-of-flight (ToF)-MS and one aliquot of each of the samples was directly analysed by MALDI-TOF-MS using the reflectron detector with an m/z range 800–4,000. The m/z values of peaks observed in samples were searched against databases of standards ( Supplementary Methods ) and diagnostic peptide markers manually identified ( Fig. 4 and Supplementary Fig. S3 ). Confirmation of the peptide markers as deriving from collagen was carried out by MS/MS sequencing of selected peptides ( Supplementary Fig. S4 and S5 ) [24] . Bone mineral analysis FEG-ESEM analysis was carried out on a Philips XL30 (Philips) equipped with an EDAX Gemini energy dispersive spectrometry system. Unprepared bone chip surfaces were analysed for surface morphology. Energy dispersive spectrometry point analyses were also completed. A standard petrographic thin section was prepared from a bone chip using only water as a cutting lubricant. The sample surface was then cleaned with deionized water and analysed via FEG-ESEM with no surface coating. Accelerating voltage was either 12 or 15 kV and chamber pressure was maintained at 0.5 torr. Take off angle was 37.1° and working distance was ~9.2 mm. How to cite this article: Rybczynski, N. et al . Mid-Pliocene warm-period deposits in the high arctic yield insight into camel evolution. Nat. Commun. 4:1550 doi: 10.1038/ncomms2516 (2013).